A platform pathway for production of 3-hydroxyacids provides a biosynthetic route to 3-hydroxy-γ-butyrolactone The replacement of petroleum feedstocks with biomass to produce platform chemicals requires the development of appropriate conversion technologies. 3-Hydroxy-γ-butyrolactone has been identified as one such chemical; however, there are no naturally occurring biosynthetic pathways for this molecule or its hydrolyzed form, 3,4-dihydroxybutyric acid. Here we design a novel pathway to produce various chiral 3-hydroxyacids, including 3,4-dihydroxybutyric acid, consisting of enzymes that condense two acyl-CoAs, stereospecifically reduce the resulting β-ketone and hydrolyze the CoA thioester to release the free acid. Acetyl-CoA serves as one substrate for the condensation reaction, whereas the second is produced intracellularly by a pathway enzyme that converts exogenously supplied organic acids. Feeding of butyrate, isobutyrate and glycolate results in the production of 3-hydroxyhexanoate, 3-hydroxy-4-methylvalerate and 3,4-dihydroxybutyric acid+3-hydroxy-γ-butyrolactone, respectively, molecules with potential uses in applications from materials to medicines. We also unexpectedly observe the condensation reaction resulting in the production of the 2,3-dihydroxybutyric acid isomer, a potential value-added monomer. Biological synthesis has emerged as a highly promising alternative to traditional organic synthesis for a variety of chemical compounds [1] , [2] . One such compound, 3-hydroxy-γ-butyrolactone (3HBL), is widely used in the pharmaceutical industry as a chiral building block for the statin class of cholesterol-reducing drugs such as Crestor and Lipitor, as well as the antibiotic Zyvox, and the antihyperlipidemic medication Zetia [3] . Other pharmaceuticals derived from 3HBL include HIV inhibitors [4] and the nutritional supplement L-carnitine [5] . 3HBL can readily be transformed into a variety of three-carbon building blocks [6] and has been listed as one of the top value-added chemicals from biomass by the US Department of Energy [7] . One impediment to broader adoption of biological systems for the production of molecules such as this is the lack of established pathways for their synthesis. There are no identified natural biochemical routes nor have engineered routes been previously reported for the biosynthesis of 3HBL or its hydrolyzed acid form, 3,4-dihydroxybutyric acid (3,4-DHBA). 3HBL is currently produced as a specialty chemical and sells at a wholesale cost of ~$450 per kg. A continuous chemical synthesis process employing high pressure hydrogenation of L-malic acid over a ruthenium-based catalyst in a fixed-bed reactor has been developed for the commercial synthesis of ( S )-3HBL at a capacity of 120 tonnes per year [8] , [9] ; however, this process employs hazardous processing conditions and expensive catalyst and purification processes. The various other chemical and chemoenzymatic routes developed for 3HBL synthesis [3] also suffer from similar disadvantages including the use of hazardous materials and processing conditions [10] , [11] , expensive starting materials, reagents and catalysts [11] , [12] , [13] , [14] , [15] , and poor yield and difficult to separate by-products [10] , [12] , [13] , [16] , driving up the cost of the product. Biosynthesis is expected to alleviate many of these problems and offer an elegant solution towards economical production of this valuable chemical; however, this requires the design of a novel biosynthetic pathway [17] , [18] . To design a pathway for the production of 3HBL, we focused on the hydrolyzed free hydroxyacid form, 3,4-DHBA. Hydroxyacids as a class are versatile, chiral compounds that contain both a carboxyl and a hydroxyl moiety, allowing for their modification into several useful derivatives [19] and making them suitable for applications in the synthesis of antibiotics [20] , β- and γ-amino acids and peptides [21] , [22] , and as chiral synthetic building blocks [23] . 3-Hydroxyacids are also naturally produced as components of polyhydroxyalkanoate (PHA) biopolymers [24] and can in turn be used to synthesize PHAs with novel properties [25] , [26] . Although many substituent monomers have been incorporated into PHAs through modulation of substrates provided in the culture medium [26] , [27] , the number of monomers produced directly from simple carbon sources is far smaller. Indeed, only 3-hydroxybutyrate (3HB) and 3-hydroxyvalerate (3HV) have been successfully produced at the gram per litre scale using enzymes of the PHA biosynthetic pathway [28] , [29] , [30] . In these reports, 3HB or 3HV synthesis begins with the condensation of two acetyl-CoA molecules or acetyl-CoA and propionyl-CoA, respectively, through the action of a thiolase enzyme (PhaA or BktB). The β-keto group is subsequently reduced to an alcohol by one of the two 3-hydroxybutyryl-CoA dehydrogenases, PhaB or Hbd, yielding the ( R ) or ( S )-enantiomer, respectively. Lastly, production of the free acid requires hydrolysis of the CoA moiety, which can be accomplished by the enzyme pair phosphotransbutyrylase (Ptb) and butyrate kinase (Buk) [28] , [31] , or by thioesterase II (TesB) [29] , [32] , [33] . TesB is capable of hydrolyzing both enantiomers of 3HB-CoA, whereas the Ptb-Buk enzyme system is specific to the ( R )-enantiomer. Unlike acetyl-CoA, propionyl-CoA is not naturally produced in E. coli in significant quantities. In Tseng et al. , [30] exogenously supplied propionate was intracellularly activated to propionyl-CoA using the previously described Ptb-Buk enzymes, known to act reversibly to produce CoA-activated compounds [31] . The successful direct production of 3HB and 3HV inspired here the adaptation of this route to produce more structurally diverse 3-hydroxyacids, especially 3,4-DHBA, thus creating a platform pathway for biological synthesis from the core enzymatic elements described above ( Fig. 1 ). The substrate range of the thiolase enzyme catalyzing the initial carbon–carbon bond-forming reaction is a key element of the pathway, and BktB exhibits broader substrate range than PhaA [34] . 3,4-DHBA synthesis using the 3-hydroxyacid pathway requires the condensation of acetyl-CoA and glycolyl-CoA; however, the ability of the BktB thiolase to catalyze this reaction was unknown. The pathway also requires the exogenous supply of glycolate, and there were no reports describing production of glycolyl-CoA from glycolate. Thus, additional CoA activation systems were investigated. These included propionyl-CoA transferase (Pct), a broad substrate specificity enzyme from Megasphaera elsdenii [35] , [36] that exchanges CoA moieties between short-chain organic acids including acetyl-CoA, and propionyl-CoA synthetase (PrpE) from Salmonella typhimurium LT2 (ref. 37 ), in addition to Ptb-Buk. We also investigated in vivo synthesis of glycolate via the glyoxylate shunt to enable direct production of 3,4-DHBA from glucose. Finally, we further explored extensibility of the pathway by feeding butyrate to determine whether longer-chain hydroxyacids could be produced and isobutyrate to examine the potential for synthesis of branched chain hydroxyacids. Although the different pathway enzyme combinations tested showed considerable differences in in vivo activities in synthesizing products from the supplied substrates, the combination consisting of Pct, BktB, PhaB and TesB was found to be most versatile and allowed synthesis of five novel products using the platform, including 3,4-DHBA, 3HBL, 2,3-dihydroxybutyric acid (2,3-DHBA), 3-hydroxyhexanoic acid (3HH) and 3-hydroxy-4-methylvaleric acid (3H4MV). 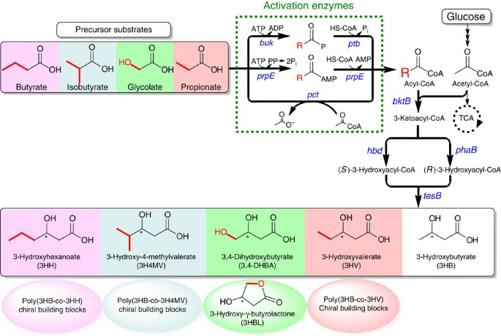Figure 1: Schematic representation of the 3-hydroxyacid pathway. Genes in blue were overexpressed, including one of the activation enzymes (encoded bypct,prpEorptb-buk), one thiolase enzyme (encoded bybktB), one of the two 3-hydroxybutyryl-CoA reductases (encoded byphaB orhbd), and one thioesterase enzyme (encoded bytesB). The carbon sources used in the system were glucose and one precursor substrate depicted enclosed by a rectangular box. The precursor substrates and their corresponding 3-hydroxyalkonoic acid products are colour coded accordingly. Figure 1: Schematic representation of the 3-hydroxyacid pathway. Genes in blue were overexpressed, including one of the activation enzymes (encoded by pct , prpE or ptb-buk ), one thiolase enzyme (encoded by bkt B), one of the two 3-hydroxybutyryl-CoA reductases (encoded by pha B or hbd ), and one thioesterase enzyme (encoded by tes B). The carbon sources used in the system were glucose and one precursor substrate depicted enclosed by a rectangular box. The precursor substrates and their corresponding 3-hydroxyalkonoic acid products are colour coded accordingly. Full size image Validation of the pathway enzymes through production of 3HV Propionate is the natural substrate for Pct and PrpE, and the ability of Ptb-Buk to activate propionate had been previously demonstrated [30] . To validate the functional expression of all pathway enzymes and to gain insights into differences in their in vivo activities and specificities, propionate and glucose were supplied to cultures of recombinant E. coli cells expressing one of the three activators ( pct , prp E or ptb- buk ), one of two 3-hydroxybutyryl-CoA reductases ( pha B or hbd ), tes B, and bkt B from their respective plasmids. 3HV was produced in all six recombinant strains, confirming functional expression of all pathway genes ( Fig. 2 ). Among the three activation enzymes, Pct resulted in the highest ( S )-3HV titres, up to 18.00±0.23 mM (2,130±27 mg l −1 ), when Hbd was utilized as the reductase (strain MG1), followed by Ptb-Buk (strain MG3) and PrpE (strain MG2). In the case of ( R )-3HV biosynthesis employing PhaB as the reductase, all three activators were generally comparable, with up to 19.65±1.81 mM (2,320±213 mg l −1 ) produced by strain MG4. The choice of reductase influenced both final 3HV titres and 3HV production rates as strains utilizing PhaB (strains MG4–6) yielded more 3HV at a faster rate than strains employing Hbd (strains MG1–3) ( Fig. 2 and Supplementary Fig. S1 ). 3HB is a by-product of the 3-hydroxyacid pathway as BktB retains high activity for the condensation of two acetyl-CoA molecules [34] to produce acetoacetyl-CoA, the natural substrate of both PhaB and Hbd. 3HB production levels were affected by the specific combination of enzymes employed ( Fig. 3 ). In all of the experiments reported here, much less 3HB was detected in strains utilizing Pct for CoA activation ( Fig. 3 , strains MG1 and MG4) compared with strains utilizing Ptb-Buk or PrpE. Pct can transfer the CoA moiety from acetyl-CoA to other short organic acids [35] . This CoA transfer should significantly reduce intracellular acetyl-CoA concentrations, making the second-order condensation of two acetyl-CoA molecules less likely than the condensation of acetyl-CoA with another acyl-CoA (a first-order reaction with respect to acetyl-CoA). Thus, strains utilizing Pct achieved the highest selectivity towards both ( S )-3HV and ( R )-3HV ( Fig. 2 ), but produced the most acetate among the three activators examined ( Fig. 3 ) as a direct consequence of the transferase reaction. 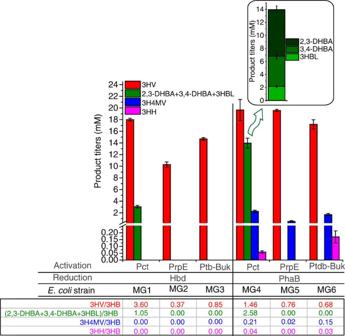Figure 2: Biosynthesis of 3-hydroxyacids through pathways with different genes and feeding of various precursors. Shake-flask production of chiral 3-hydroxyacids at 72 h. The various recombinant strains are described inTable 1. Production of 3HV (red bars), 2,3-DHBA+3,4-DHBA+3HBL (green bars), 3H4MV (blue bars) and 3HH (pink bars) was achieved with supplementation of propionate, glycolate, isobutyrate and butyrate, respectively, in addition to glucose. Data are presented as the mean±s.d. (n=3). The specific activation enzymes and reductases used in each pathway are shown on thexaxis. Product selectivity, defined as the molar ratio of the quantity of desired 3-hydroxyacid to the quantity of concomitant product of 3HB, is shown below thexaxis. Inset shows breakdown of 2,3-DHBA, 3,4-DHBA and 3-HBL synthesized by strain MG4. 2,3-DHBA was below the limit of quantitation for strain MG1.Supplementary Table S1shows the product yields on the supplied substrates. Figure 2: Biosynthesis of 3-hydroxyacids through pathways with different genes and feeding of various precursors. Shake-flask production of chiral 3-hydroxyacids at 72 h. The various recombinant strains are described in Table 1 . Production of 3HV (red bars), 2,3-DHBA+3,4-DHBA+3HBL (green bars), 3H4MV (blue bars) and 3HH (pink bars) was achieved with supplementation of propionate, glycolate, isobutyrate and butyrate, respectively, in addition to glucose. Data are presented as the mean±s.d. ( n =3). The specific activation enzymes and reductases used in each pathway are shown on the x axis. Product selectivity, defined as the molar ratio of the quantity of desired 3-hydroxyacid to the quantity of concomitant product of 3HB, is shown below the x axis. Inset shows breakdown of 2,3-DHBA, 3,4-DHBA and 3-HBL synthesized by strain MG4. 2,3-DHBA was below the limit of quantitation for strain MG1. Supplementary Table S1 shows the product yields on the supplied substrates. 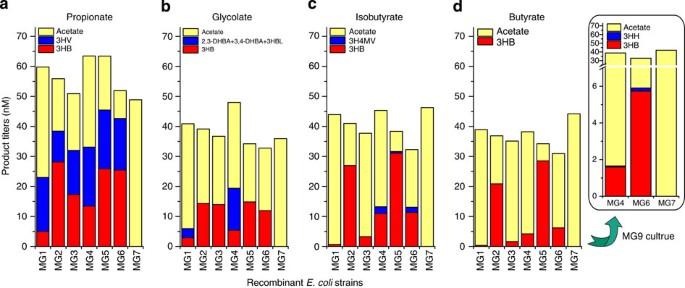Figure 3: Metabolite profile of the various recombinantE. colicultures supplemented with various precursors. Metabolite profile of major products, including the desired 3-hydroxyacid, 3HB and acetate, from various combinations of pathway enzymes supplemented with various precursor substrates ((a) propionate; (b) glycolate; (c) isobutyrate; and (d) butyrate). The specific recombinant strains used are shown on thexaxis (Table 1). As mentioned in theMethods, 3HH cannot be resolved during HPLC separation from one of the LB peaks; hence 3HH titres were not plotted for LB cultures ind. The inset indshows titres for M9 cultures of the two 3HH producing strains MG4 and MG6 and the control strain MG7. Full size image Figure 3: Metabolite profile of the various recombinant E. coli cultures supplemented with various precursors. Metabolite profile of major products, including the desired 3-hydroxyacid, 3HB and acetate, from various combinations of pathway enzymes supplemented with various precursor substrates (( a ) propionate; ( b ) glycolate; ( c ) isobutyrate; and ( d ) butyrate). The specific recombinant strains used are shown on the x axis ( Table 1 ). As mentioned in the Methods , 3HH cannot be resolved during HPLC separation from one of the LB peaks; hence 3HH titres were not plotted for LB cultures in d . The inset in d shows titres for M9 cultures of the two 3HH producing strains MG4 and MG6 and the control strain MG7. Full size image Production of 3,4-DHBA and 3HBL from glucose and glycolate The platform pathway was designed to produce 3,4-DHBA from glycolate as a precursor ( Fig. 1 ). In cultures supplemented with glycolate and glucose, only the pct -expressing strains, MG1 and MG4, produced 3,4-DHBA, whereas strains expressing the activators prpE and ptb-buk only synthesized 3HB and acetate ( Figs 2 and 3 ). Unexpectedly, these cultures also produced small quantities of 3HBL. The lactone could be formed either due to direct spontaneous lactonization of the 3,4-dihydroxybutyryl-CoA intermediate or from free 3,4-DHBA upon equilibration under the culture conditions. If the former were true, then elimination of TesB from the pathway should result in increased 3HBL synthesis. In strains not expressing the tes B gene, 52% more 3HBL and 96% less 3,4-DHBA was produced ( Supplementary Fig. S2 ). Moreover, equilibration of 3,4-DHBA standards under final culture conditions (pH~5.5, 30 °C) did not result in detectable lactonization of 3,4-DHBA to 3HBL. These results support the hypothesis that 3HBL was produced by the direct cyclization of the 3,4-dihydroxybutyryl-CoA intermediate. A similar spontaneous lactonization is hypothesized to result in the synthesis of γ-butyrolactone from 4-hydroxybutyryl-CoA [38] . The identity of 3,4-DHBA and 3HBL was confirmed through high-performance liquid chromatography (HPLC) and HPLC/mass spectrometry (MS) analysis (see Methods ). Strain MG4, expressing pct and phaB in addition to bktB and tesB , synthesized up to 4.62±0.33 mM (555±52 mg l −1 ) of 3,4-DHBA and 2.17±0.15 mM (221±15 mg l −1 ) of 3HBL. The total 3,4-DHBA and 3HBL titres estimated on a molar basis were about two-fold higher with PhaB as a reductase than with Hbd ( Fig. 2 ), indicating limitations associated with the activity of Hbd towards the non-natural substrate 4-hydroxy-3-ketobutyryl-CoA. Investigating a pathway side product: synthesis of 2,3-DHBA In addition to 3,4-DHBA, strains MG1 and MG4 synthesized a second species that co-eluted with 3,4-DHBA during HPLC analysis ( Supplementary Fig. S3 ). This species eluted immediately adjacent to the 3,4-DHBA ammonium adduct and was detected at the same m/z ratio of 138.1 during HPLC/MS analysis ( Supplementary Fig. S4 ). In the absence of glycolate or the pathway enzymes, the product was not detected, indicating that the species was a structural isomer generated by the platform pathway. 2,3-DHBA was one possible isomeric product, identical in mass to 3,4-DHBA, that we hypothesized could be formed through an alternative Claisen condensation reaction [39] catalyzed by BktB [40] . The condensation reaction between glycolyl-CoA and acetyl-CoA that results in the synthesis of 3,4-DHBA involves abstraction of an α-proton from acetyl-CoA to generate a carbanion that initiates the formation of the carbon–carbon bond in the 4-hydroxy-3-ketobutyryl-CoA intermediate ( Fig. 4a and Supplementary Fig. S5 ). Alternatively, the abstraction of an α-proton from glycolyl-CoA ( Fig. 4b and Supplementary Fig. S6 ) is expected to result in the synthesis of 2,3-DHBA via the 2-hydroxy-3-ketobutyryl-CoA intermediate. The absence of a commercially available standard for 2,3-DHBA prevented the direct confirmation of this hypothesis using HPLC/MS analysis. Thus, we used labelled glycolate in which both of the hydrogen atoms on the α-carbon were replaced with deuterium to investigate further ( Fig. 4c ). As expected, a peak corresponding to the doubly deuterated 3,4-DHBA ammonium adduct ( Fig. 4c ) was observed at an m/z ratio of 140.1 that coincided with the peak for the unlabelled 3,4-DHBA standard detected at an m/z of 138.1, confirming 3,4-DHBA synthesis in strain MG4 ( Supplementary Fig. S4 ). Further, a peak corresponding to the unknown species was detected at an m/z of 139.1. The loss of 1 mass unit relative to the labelled 3,4-DHBA ammonium adduct was consistent with the mechanism for formation of 2,3-DHBA by the alternative Claisen condensation reaction ( Fig. 4b and Supplementary Fig. S6 ). The 2,3-DHBA isomer was subsequently confirmed via nuclear magnetic resonance analysis (see Supplementary Methods and Supplementary Fig. S7 ). 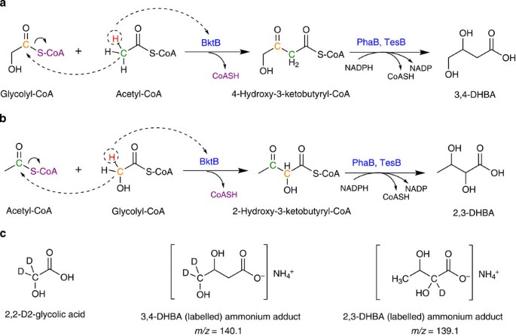Figure 4: Synthesis of DHBA isomers via the Claisen condensation reaction. (a) Formation of 3,4-DHBA; (b) formation of 2,3-DHBA; (c) structures of the deuterium-labelled glycolate, 3,4-DHBA and 2,3-DHBA ammonium adducts detected via HPLC/MS. Encircled and highlighted in red are the α-protons abstracted by the enzyme for the generation of the carbanion responsible for the carbon–carbon bond forming nucleophilic substitution reaction in each case (detailed mechanism depicted inSupplementary Figs S5 and S6). Also highlighted are the respective carbon atoms from each substrate involved in the carbon–carbon bond formation. Figure 4: Synthesis of DHBA isomers via the Claisen condensation reaction. ( a ) Formation of 3,4-DHBA; ( b ) formation of 2,3-DHBA; ( c ) structures of the deuterium-labelled glycolate, 3,4-DHBA and 2,3-DHBA ammonium adducts detected via HPLC/MS. Encircled and highlighted in red are the α-protons abstracted by the enzyme for the generation of the carbanion responsible for the carbon–carbon bond forming nucleophilic substitution reaction in each case (detailed mechanism depicted in Supplementary Figs S5 and S6 ). Also highlighted are the respective carbon atoms from each substrate involved in the carbon–carbon bond formation. Full size image MG4 supplied with unlabelled glycolate was estimated to have synthesized 7.17± 0.54 mM (860±65 mg l −1 ) of 2,3-DHBA ( Fig. 2 ). These titres were comparable to the total of 3,4-DHBA and 3HBL (about 6.8 mM) produced in the same cultures, and suggest a roughly equal selectivity of BktB towards both isomers. Although MG1 cultures also synthesized small quantities of 2,3-DHBA, these were too small to be quantified accurately using HPLC. 3,4-DHBA to 3HBL conversion by acid treatment It is well documented that lactonization is acid-catalyzed [41] ; hence, the equilibrium between 3,4-DHBA and 3HBL was expected to be governed by pH, amongst other factors. Overnight acid treatment of 3,4-DHBA standards in LB with 6 N hydrochloric acid at 37 °C resulted in a progressive shift in the equilibrium towards 3HBL with decreasing pH, with a maximum K of 1.9 ( K =(3HBL)/(DHBA)) at a pH close to 0.7 ( Supplementary Fig. S8 ). Acid treatment of culture supernatants from strains MG1 and MG4 allowed effective conversion of 3,4-DHBA to 3HBL. Strain MG4 expressing the pct-phaB activator–reductase combination showed the highest post-acid treatment 3HBL titres of 4.53±0.33 mM (462±35 mg l −1 ) and corresponding 3,4-DHBA titres of 2.27±0.17 mM (272±20 mg l −1 ) ( Fig. 5 ). 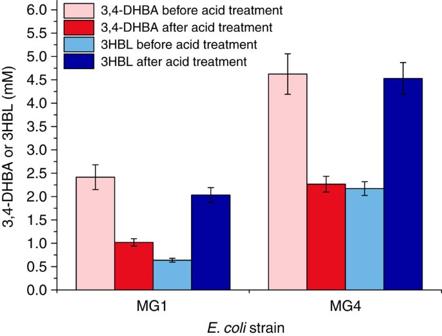Figure 5: 3,4-DHBA and 3HBL titres before and after acid treatment. Culture supernatants from strains MG1 and MG4 were subjected to overnight treatment with 50 mM hydrochloric acid at 37 °C, allowing for effective conversion of 3,4-DHBA to 3HBL. Bars in light colours represent samples before acid treatment, whereas bars in dark colours represent samples after acid treatment. Figure 5: 3,4-DHBA and 3HBL titres before and after acid treatment. Culture supernatants from strains MG1 and MG4 were subjected to overnight treatment with 50 mM hydrochloric acid at 37 °C, allowing for effective conversion of 3,4-DHBA to 3HBL. Bars in light colours represent samples before acid treatment, whereas bars in dark colours represent samples after acid treatment. Full size image Direct production of DHBA/3HBL from glucose Glycolate can be directly synthesized in E. coli through the reduction of glyoxylate, mediated by the endogenous glyoxylate reductase (YcdW). However, the glyoxylate shunt ( Supplementary Fig. S9 ) is heavily regulated and is typically repressed during growth on glucose or other carbon sources that are easily metabolized [42] . The glyoxylate shunt is regulated by the phosphorylation state of isocitrate dehydrogenase (Idh), which is both phosphorylated and de-phosphorylated by Idh kinase/phosphatase (AceK). Isocitrate lyase (AceA) catalyzes the cleavage of isocitrate to glyoxylate and succinate. We first examined the production of glycolate directly from glucose, using a minimal (M9) medium to limit the available carbon sources and induce the glyoxylate shunt. Overexpression of ycdW, aceA and aceK from the plasmid pHHD/ycdW-aceA-aceK in strain MG0-GP resulted in 1.4 g l −1 glycolate produced from 10 g l −1 glucose. Transformation of this strain with plasmids expressing pct , bktB , phaB and tesB (strain MG4-GDHP) resulted in the production of 3.79±0.72 mM (456±87 mg l −1 ) of 2,3-DHBA, 3.97±0.57 mM (476±67 mg l −1 ) of 3,4-DHBA and 1.85±0.26 mM (189±26 mg l −1 ) of 3HBL, from 10 g l −1 glucose as a sole carbon source. Production of six carbon hydroxyacids To explore the potential of the pathway to incorporate longer chain, aliphatic substrates, isobutyrate and butyrate were supplied to the culture medium to investigate the production of the six carbon isomers 3H4MV and 3HH, respectively. Although DHBA synthesis was only observed with Pct, all three CoA activation systems resulted in the production of 3H4MV, and all except PrpE could produce 3HH ( Figs 2 and 3 , strains MG4–6). However, both 3H4MV and 3HH were detected only with the PhaB reductase ( Figs 2 and 3 , strains MG4–6). For 3H4MV, a fourth CoA-activation system was tested, namely, Bacillus subtilis Ptb-Buk. This system was chosen because of its association with genes involved in branched-chain fatty acid synthesis, suggesting a preference for branched acids such as isobutyrate [43] . The B. subtilis Ptb-Buk enzyme system resulted in 3H4MV titres comparable to those obtained with the Clostridium acetobutylicum homologues, but produced more 3HB and less acetate ( Supplementary Fig. S10 ). This suggests that the two Ptb-Buk homologues may be equally efficient in activating isobutyrate, but the B. subtilis pair has lower activity with acetyl-CoA resulting in lower acetate and higher 3HB, as the increased acetyl-CoA pool would favour 3HB synthesis. Overall, 3H4MV titres were observed up to 2.27±0.18 mM (300±25 mg l −1 ) in strain MG4 and 3HH titres up to 0.170±0.04 mM (22.5±5.9 mg l −1 ) were achieved in strain MG6. Biological synthesis of chemical compounds is an attractive option that is in part limited by the availability of synthetic pathways for molecules of interest. Expanding this capacity thus requires the de novo design of biosynthetic routes. This work represents the first report of a platform pathway for 3-hydroxyacid synthesis that results in the complete biological production of the value-added compounds 3,4-DHBA and 3HBL. A key enzyme in the platform pathway developed is the thiolase, BktB, which catalyzes the Claisen condensation. Carbon–carbon bond forming chemistry provides a unique way to extend beyond naturally occurring backbones to generate a wider array of compounds. In most other examples of pathway design for targeted molecule production, carbon–carbon bonds are either broken through decarboxylation (for example, production of 1,2,4-butanetriol from pentose sugars [44] ; fusel alcohols from amino acid precursors [45] ) or the carbon chain length is already set through a naturally occurring metabolic intermediate (for example, 3-hydroxypropionic acid from pyruvate or alanine [46] ; 1,4-butanediol from succinate or succinyl semialdehyde through decarboxylation of alpha-ketoglutarate [38] ). An ability to set carbon skeletons with unnatural substrates represents an entirely new opportunity to envision and achieve targeted microbial synthesis of value-added compounds. A recently published study reports carbon chain elongation for targeted production of the unnatural branched alcohol, 3-methyl-1-pentanol; however, eight other alcohols were produced as by-products [47] . Thus, our ability to produce the targeted compounds through the formation of a new carbon–carbon bond while producing only two related analogs (2,3-DHBA and 3HB) represents a significant achievement. The platform pathway developed herein has the flexibility to produce various molecules based on the precursors supplied (either exogenously or endogenously) and to generate different stereoisomers based on the choice of reductase employed. It is well documented that PhaB results exclusively in ( R )-3-hydroxyacids while Hbd results in the ( S ) stereoisomers [33] , [48] . This phenomenon was experimentally verified in pathways producing both 3HB [29] and 3HV [30] . Because 3,4-DHBA has a hydroxyl group in the δ-position that changes the stereochemical priority of the different atoms of the molecule about its stereocenter, the stereochemistry of 3,4-DHBA formed by PhaB should be ( S )-3,4-DHBA while that formed by Hbd should be ( R )-3,4-DHBA. PhaB results in significantly higher titres, and fortunately, the ( S ) stereoisomer is predominately used in the production of pharmaceuticals and high-value compounds [3] . Identification and screening of hbd homologues could identify a reductase with identical stereochemical preference but with an increased substrate tolerance for the production of ( R )-3,4-DHBA and ( R )-3HBL. A notable finding in this work was the observation of the alternative Claisen condensation reaction to yield the 2,3-DHBA isomer. As the reaction mechanism requires the abstraction of an α-proton to initiate nucleophilic attack, we do not expect all molecular pairs to be equally likely to form both isomers. Indeed, our inability to observe any alternative products in the synthesis of 3HV is consistent with a previous report that found no activity with a BktB homologue from Zoogloea ramigera (51% identity/68% similarity) in the thiolytic direction with the branched 2-methylacetoacetyl-CoA isomer of β-ketovaleryl-CoA [40] . The unexpected production of 2,3-DHBA is an exciting development because of the implication for other molecular structures that could be formed using substrates with sufficiently electronegative α-protons. In addition, the compound is of specific interest because of its utility as a potential commercial target. Indeed, the 2,3-isomer is attractive as a monomer for use in the synthesis of hyperbranched polymers [49] . Although our achievable titres of nearly 800 mg l −1 ( S )-3,4-DHBA/3HBL from glucose and glycolate and ~650 mg l −1 from glucose as a sole carbon source certainly require improvement for large-scale production, these values are extremely promising as the first demonstration of engineered synthesis in comparison to other engineered pathways that rely on carbon–carbon bond forming reactions. Khosla and colleagues [50] reported titres of ~25 mg l −1 in the initial reconstruction of polyketide synthesis in E.coli, while the Keasling group obtained maximum amorphadiene titres of 112 mg l −1 in the first reported synthesis in an engineered organism [51] . These low titres were observed in spite of the availability of natural pathways to produce the target molecules. The latter example is especially encouraging given more recent reports of 27.4 g l −1 amorphadiene produced in 2-L fed-batch reactors [52] . Indeed, we anticipate that production of ( S )-3,4-DHBA/3-HBL at comparable titres can result in a substantial reduction in cost of goods for high-value applications such as pharmaceutical synthesis. Taken together, the initial findings of novel molecules produced here point to three main avenues for greatly enhancing the potential of this pathway to launch new commercial bio-products. First, the full potential of the wild-type enzymes remains unknown from the small subset of substrates that were screened. The broad substrate range of the thiolase for catalyzing carbon–carbon bond-forming reactions, an essential first step, enables one to envision a wide array of novel compounds that could be produced and subsequently transformed into products ranging from medicines to materials. Further characterization of the promiscuous CoA-activating enzyme Pct may also lead to the use of this enzyme in additional novel pathways that rely on CoA-containing compounds, including those involved in fatty acid β-oxidation, Clostridial n -butanol biosynthesis, and the mevalonate-dependent isoprenoid pathway. Second, improving upon the activities of the pathway enzymes, either through screening for more active homologues or through protein engineering, should result in both broader substrate range and higher production titres. Of particular interest is protein engineering to influence product formation [53] , for example, to preference 3,4- over 2,3-DHBA synthesis or to accelerate the alternative Claisen condensation, producing novel branched or α-substituted molecules. Finally, production strains for hydroxyacid synthesis can be further engineered to produce pathway substrates endogenously, as demonstrated here for the production of DHBA and 3HBL from glucose and previously to produce 3HV from glucose or glycerol as the sole carbon source [30] . Intracellular production of pathway substrates would mitigate the cost and/or toxicity associated with the secondary carbon sources as well as eliminate the need for substrate transport across the cellular envelope, potentially accelerating production. Each of these approaches has the potential to further enhance the platform pathway we present here as an efficient and sustainable avenue for the production of value-added biochemicals. Strains and plasmids Strains and plasmids used in this study are listed in Table 1 . E. coli DH10B (Invitrogen, Carlsbad, CA) and ElectroTen-Blue (Stratagene, La Jolla, CA) were used for transformation of cloning reactions and propagation of all plasmids. E. coli MG1655(DE3 Δ end A Δ rec A) was described previously (as strain HCT10 (ref. 30 )) and was used as the production host for hydroxyacid synthesis, as well as endogenous glycolate synthesis. Table 1 E. coli strains and plasmids used in the 3-hydroxyacid pathway. Full size table Genes from C. acetobutylicum ATCC 824 ( ptb-buk and hbd ), Cupriavidus necator H16, formerly known as Ralstonia eutropha H16 ( bkt B and pha B), E. coli K-12 ( tes B, ycd W, and ace A- ace K), M. elsdenii ( pct ), S. typhimurium LT2 ( prp E) and B. subtilis 3610 ( ptb and buk ) were obtained by PCR using genomic DNA (gDNA) templates. All gDNAs were prepared using the Wizard Genomic DNA Purification Kit (Promega, Madison, WI). Custom oligonucleotides (primers) were purchased for all PCR amplifications (Sigma-Genosys, St Louis, MO) as listed in Supplementary Table S2 . In all cases, Phusion High Fidelity DNA polymerase (Finnzymes, Espoo, Finland) was used for DNA amplification. Restriction enzymes and T4 DNA ligase were purchased from New England Biolabs (Ipswich, MA). Recombinant DNA techniques were performed according to standard procedures. Two co-replicable vectors, pETDuet-1 and pCDFDuet-1 (Novagen, Darmstadt, Germany), were used for construction of the 3-hydroxyacid pathway plasmids. Plasmid pHHD was constructed from pKVS45 and enables expression of genes under the control of a tetracycline inducible promoter (see Supplementary Methods ). This plasmid is compatible with the Duet vectors. The sites used for cloning the genes are underlined in Supplementary Table S2 . PCR products were digested with the appropriate restriction enzymes and ligated directly into similarly digested vectors. The ptb-buk fragment was generated by Eco RI and Not I digestion of pCDF-PB [29] . The B. subtilis ptb and buk genes were cloned into an artificial operon using splicing by overlap extension PCR [54] , [55] to mimic the natural C. acetobutylicum ptb-buk operon. The E. coli genes ycdW , aceA and aceK were similarly cloned into an artificial operon to mimic the structure of the natural aceB-aceA-aceK operon in E. coli , with the ycdW gene replacing aceB (see Supplementary Methods ). Ligation reactions using pETDuet-1 and pHHD as vectors were used to transform E. coli DH10B, whereas ligations using pCDFDuet-1 were used to transform E. coli ElectroTen-Blue. One thiolase ( bkt B) and one of the two 3-hydroxybutyryl-CoA reductases ( pha B and hbd ) were cloned into pETDuet-1. The pCDFDuet-based plasmids contained one of the four CoA-activation genes ( pct , ptb-buk , ptb-buk ( Bs ) and prp E) and one thioesterase ( tes B). The artificial operon ycdW-aceA-aceK was ligated into pHHD for construction of the plasmid pHHD/ycdW-aceA-aceK that allows expression of enzymes for endogenous glycolate synthesis upon induction with anhydrotetracycline (aTc). All constructs were confirmed to be correct by restriction enzyme digestion and nucleotide sequencing. Once all plasmids were constructed, one pETDuet-based plasmid and one pCDFDuet-based plasmid were used to co-transform E. coli MG1655(DE3)Δ endA Δ recA (MG0) to create hydroxyacid production strains. For endogenous synthesis of glycolate, strain MG0-GP was constructed by transforming MG0 with pHHD/ycdW-aceA-aceK. MG4 was transformed with pHHD/ycdW-aceA-aceK to construct strain MG4-GDHP to study the direct synthesis of glycolate, the two DHBAs and 3-HBL from glucose as a sole carbon source. Culture conditions Seed cultures of the recombinant E. coli strains ( Table 1 ) were grown in LB medium at 30 °C overnight, and were used to inoculate 50 ml LB medium supplemented with 10 g l −1 glucose at an inoculation volume of 2% in 250 ml flasks. Owing to HPLC peak overlapping between 3HH and LB components, 3HH biosynthesis was conducted in M9 minimal medium supplemented with 10 g l −1 glucose, where seed cultures were washed and re-suspended in M9 minimal medium before inoculation. The shake flask cultures were then incubated at 30 °C on a rotary shaker at 250 r.p.m. Once the cells reached mid-exponential phase (when OD 600 reached 0.8–1.0), cultures were supplemented (final concentrations in parentheses) with isopropyl-β- D -thiogalactoside (IPTG) (1 mM) for induction of gene expression and one of the precursor substrates: neutralized propionate (15 mM), butyrate (15 mM), isobutyrate (15 mM) and glycolate (40 mM). In all cases, culture medium was supplemented with 50 mg l −1 ampicillin and 25 mg l −1 streptomycin to provide selective pressure for plasmid maintenance. The direct synthesis of glycolate, 2,3-DHBA, 3,4-DHBA and 3-HBL from glucose as a sole carbon source in strains MG0-GP and MG4-GDHP was also conducted in M9 minimal medium to promote glycolate synthesis via the glyoxylate shunt. MG0-GP cultures were supplemented with 50 mg l −1 kanamycin and induced with aTc (250 ng ml −1 ) while MG4-GDHP cultures were supplemented with ampicillin (50 mg l −1 ), streptomycin (50 mg l −1 ) and kanamycin (30 mg l −1 ) and simultaneously induced with aTc (250 ng ml −1 ) and IPTG (100 μM) in mid-exponential phase. One millilitre of culture was withdrawn every 24 h for up to 96 h for HPLC and HPLC/MS analysis. Titres of 3-hydroxyacids reached a plateau at 72 h and there was essentially no difference in the titres between 72 and 96 h; accordingly, only the peak titres observed at 72 h were reported. In general, experiments are performed in triplicates, and data are presented as the averages and s.d. of the results. Metabolite analysis Culture samples were pelleted by centrifugation and aqueous supernatant collected for HPLC analysis using an Agilent 1200 series instrument with a refractive index detector (RID). Analytes were separated using an Aminex HPX-87H anion-exchange column (Bio-Rad Laboratories, Hercules, CA) and a 5 mM H 2 SO 4 mobile phase. Glucose, propionate, butyrate, isobutyrate, glycolate, acetate, 3HB, 3HV, 3-hydroxyhexanoate and ( S )-3HBL were quantified using commercial standards by linear interpolation from calibration of external standards. Owing to the absence of a commercially available standard, the 3,4-DHBA standard used for HPLC analysis was prepared from ( S )-3HBL by saponification at 37 °C for 3 h at pH>10 using 10 N sodium hydroxide. Complete conversion of ( S )-3HBL to ( S )-3,4-DHBA (as confirmed by disappearance of the 3HBL peak on the HPLC time trace) was observed during this treatment. In addition, 3,4-DHBA and 2,3-DHBA synthesis was also confirmed using HPLC/MS analysis on an Agilent 1100 series instrument equipped with 6120 Quadrapole MS with multi-mode source and an Aminex HPX-87H column with 25 mM ammonium formate as the mobile phase. The ammonium adduct of 3,4-DHBA was detected at an m/z ratio of 138.1 to confirm 3,4-DHBA synthesis in the samples ( Supplementary Fig. S4 ). The ammonium adduct of deuterium-labelled 3,4-DHBA formed from deuterium-labelled 2,2-D2-glycolic acid was detected at an m/z ratio of 140.1 while that of deuterium labelled 2,3-DHBA was detected at an m/z ratio of 139.1. Preparative chromatography was used to co-purify 2,3-DHBA and 3,4-DHBA from the culture supernatants (see Supplementary Methods ). The identity of 3,4-DHBA and 2,3-DHBA was confirmed via 1 H, 13 C, heteronuclear single quantum coherence, and heteronuclear multiple bond correlation NMR using a Varian 500 MHz spectrometer ( Supplementary Fig. S7 ). Owing to co-elution of 2,3-DHBA with 3,4-DHBA during separation of culture supernatants on the Aminex Column during HPLC analysis, the 3,4-DHBA and 2,3-DHBA titres were estimated indirectly as described in the Supplementary Information ( Supplementary Methods ). 3H4MV was analyzed using HPLC/MS as a commercial standard was not available. A Zorbax SB-Aq alkyl bonded phase column (Agilent Technologies, Wilmington, DE) with a 25 mM, pH 3 ammonium formate mobile phase was used to separate 3H4MV for detection with an Agilent 1100 series instrument equipped with either RID or 6120 Quadrapole MS with multi-mode source. The commercial 3HH isomer was used with RID to estimate the concentration of 3H4MV in supernatant samples. The ammonium adducts of 3H4MV and 3HH were detected at an m/z of +150.1 to confirm the presence of the branched isomer ( Supplementary Fig. S11 ). How to cite this article: Martin, C. H. et al. A platform pathway for production of 3-hydroxyacids provides a biosynthetic route to 3-hydroxy-γ-butyrolactone. Nat. Commun. 4:1414 doi: 10.1038/ncomms2418 (2013).